Monolithic focused reference beam X-ray holography Fourier transform holography is a highly efficient and robust imaging method, suitable for single-shot imaging at coherent X-ray sources. In its common implementation, the image contrast is limited by the reference signal generated by a small pinhole aperture. Increased pinhole diameters improve the signal, whereas the resolution is diminished. Here we report a new concept to decouple the spatial resolution from the image contrast by employing a Fresnel zone plate to provide the reference beam. Superimposed on-axis images of distinct foci are separated with a novel algorithm. Our method is insensitive to mechanical drift or vibrations and allows for long integration times common at low-flux facilities like high harmonic generation sources. The application of monolithic focused reference beams improves the efficiency of high-resolution X-ray Fourier transform holography beyond all present approaches and paves the path towards sub-10 nm single-shot X-ray imaging. The development of highly efficient and robust X-ray imaging methods is of particular interest for single-shot applications [1] , [2] , [3] , [4] , [5] , in which all information has to be encoded by the limited number of photons of a single femtosecond X-ray pulse, requiring outstanding efficiency of the method used. One of the few approaches that fulfil such requirements is X-ray Fourier transform holography (FTH) [6] , [7] . In FTH, the far-field scattering pattern of a specimen is recorded on a two-dimensional detector. The phase information is encoded in the interference of the scattered beam with an unperturbed reference beam, forming the hologram [1] , [6] , [8] , [9] , [10] , [11] , [12] . With an off-axis reference beam originating ideally from a point source in the object plane, the image is reconstructed by an inverse Fourier transform of the hologram as the cross-correlation of the specimen with the reference transmission function [13] . Since the FTH scattering geometry allows for recording large scattering angles, the resolution is typically limited by the spatial extent of the reference source while the image contrast is determined by the photon flux in the reference beam. (We here consider the typical case in high-resolution imaging that the reference wave is significantly weaker than the object wave and hence the limiting factor for the hologram fringe visibility). In addition, the number of pixels of the detector defines a maximum lateral size of the combined object and reference structures of the sample for a given spatial resolution [13] . In the most common implementation of FTH, the reference wave originates from a small pinhole aperture fabricated into an X-ray-opaque metal film adjacent to an object aperture that defines the field of view [6] . This integrated, monolithic design is the reason for the remarkable stability of mask-based FTH against drift and vibration of the set-up. In conjunction with the flexibility in sample environments afforded by the absence of further optical elements in the vicinity of the sample and the robust and unambiguous image reconstruction process, this approach is applied—beyond method development—for example, in material science research of magnetic nanostructures [7] , [14] , [15] . The drawback of point-like apertures generating reference waves is the entanglement of spatial resolution and contrast in the reconstruction. If the reference diameter is decreased, the resolution limit will scale linearly with the reference size while the reference signal strength, and ultimately the image contrast, is reduced quadratically. A high-resolution FTH imaging experiment is therefore commonly designed as a compromise between the desired resolution and the required reference signal. As long as the reference signal exceeds the detector’s noise level, the decrease in flux through an ever smaller reference could in principle be accounted for by extending exposure times up to a certain practical limit. However, resolution limits as reported for Fresnel zone plate (FZP)-based X-ray microscopy [16] have not been achieved for FTH using reference pinholes with high aspect ratio up to now. Moreover, for the growing class of dynamic studies relying on femtosecond X-ray pulses, the signal has to be collected from a limited number of photons [3] , [4] , [5] , [7] . It has been demonstrated that the image contrast can be improved in a monolithic approach by using multiple reference pinholes. The final image is then retrieved either by the sum of all independent reconstructions [10] , [17] or by a Hadamard convolution if the references have been arranged in a so-called uniform redundant array [1] . However, the number of pinholes required to keep the total reference beam intensity constant while decreasing the pinhole diameters scales with the inverse square of the spatial resolution. At the same time, the space available for the object-reference arrangement shrinks according to the detector specifications [13] . With present-day nanofabrication tools, the density of pinholes is insufficient to prepare an adequate number of such reference holes in sub-10 nm spatial resolution-imaging experiments. To avoid the dilemma of entanglement between resolution and contrast in the object reconstruction, the reference beam cannot be provided by pinhole apertures. Following the original idea of holography as proposed by Denis Gabor [18] , we have replaced the pinhole aperture by an X-ray lens, realized by a FZP. The flux in the FZP focus, that is, the intensity integrated over the size of the focus, which determines the contrast in the image reconstruction, is proportional to the FZP’s diameter D , whereas the focal spot size is defined by the outermost zone width Δ r (ref. 19 ). The FZP diameter D can easily be adjusted by altering the number of zones N such that ideally the flux through the FZP approximates the flux through the object. For conventional lens-based imaging techniques like X-ray microscopy, the small focal length f of high-resolution FZPs complicates sample positioning and limits the space available for additional instruments in the vicinity of the sample. Similar to conventional soft-X-ray FTH [6] , and contrary to previous off-axis and in-line holography experiments employing FZPs [8] , [9] , [20] , [21] , we have fabricated the FZP directly into the integrated sample-mask structure, retaining the mechanical stability and flexibility with regard to sample environments of the FTH set-up. Particularly with respect to application scenarios at modern femtosecond X-ray sources such as high harmonic generation and free-electron laser sources, our method overcomes crucial limitations of previous implementations. First, our method is fully compatible with time-resolved optical pumping experiments as the reference FZP does not occupy the vicinity upstream of the sample and, second, owing to the monolithically integrated design, the resolution is not affected by pointing instabilities that are common at those sources [9] . The high stability of our implementation allows for very long integration times over many thousand X-ray pulses as required at photon-limited sources like high harmonic generation to achieve high spatial resolution. Focused reference beam concept For the integrated mask design, the FZP focal length can be chosen as a free parameter (since no mechanical restrictions need to be considered), facilitating the flexible adjustment of the remaining FZP parameters. In contrast to conventional FTH reconstructions, which yield a focused image of the object exit wave in the mask plane, the reconstruction of the FZP-generated hologram describes the object exit wave field in the FZP focal planes, as sketched in Fig. 1 . The geometric separation of the FZP focus and the specimen along the optical axis can be accounted for by numerically propagating the reconstructed object wave from the focal plane to the sample plane [22] , [23] , [24] . A binary FZP focuses up to 10% of the transmitted light into each first-order focus at a focal distance ± f (ref. 19 ) and significant further efficiency increase is possible in more refined FZP schemes [25] . The remaining light is either transmitted unperturbed (zeroth order) or focused at smaller focal distances f / n (where n is the FZP diffraction order that can take any odd positive or negative integer value). In our holographic imaging scheme, all FZP foci give rise to independent (defocused) images and by using the appropriate numerical propagation length ( p=−f / n ) each image can be brought into focus. The desired image is obtained as the cross-correlation between the specimen exit wave and the FZP focus beam profile. Depending on the propagation direction, the obtained image originates either from the real ( n >0) or the virtual focal plane ( n <0). Focused images related to different foci can be added together to further improve the signal-to-noise ratio. For an ideal binary FZP, the reference signal therefore approaches 25% of the flux incident on the FZP if many diffraction orders are considered for the reconstruction. In this case, the efficiency even approximates that of a perfect lens if FZPs with phase-shifting zones are utilized [26] . In contrast to FZP-based full-field imaging, our method capitalizes exclusively on the FZP focal spot generated on-axis. Off-axis aberrations such as astigmatism and field curvature observed for FZPs with a low number of zones [27] do not have to be considered. We can therefore use simple and disposable FZPs with very few zones, which make our method particularly suitable for destructive single-shot studies at free-electron laser facilities. Note that a correction of the hologram distortion due to a flat area detector may have to be considered for high scattering angles [28] . 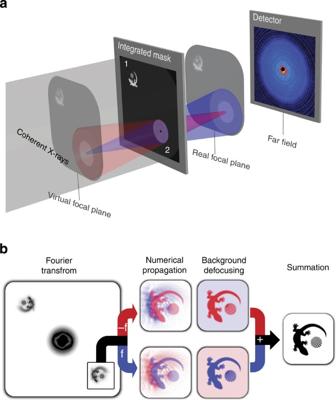Figure 1: Monolithic focused reference beam holography scheme. (a) Experimental geometry and imaging scheme for FTH with the FZP first-order foci. The integrated mask contains both the object (1) to be imaged as well as a FZP (2). Positive and negative FZP diffraction orders are focused in a real and a virtual focal plane, respectively. The reference beams corresponding to these focal planes encode the phase information of the object beam by interference. In each focal plane, the object exit wave appears to be defocused by the FZP focal lengthf. (b) The Fourier transform of the recorded hologram is depicted on the left side, containing a defocused holographic object reconstruction (black box). A focused reconstruction can be obtained by numerically propagating the defocused reconstruction by ±f, yielding an in-focus image that is superimposed by the reconstruction of the opposite focal plane (middle). After defocusing the undesired opposite focal-plane contributions for both FZP diffraction orders, virtual and real-image reconstructions can be added to further improve the signal (right). Figure 1: Monolithic focused reference beam holography scheme. ( a ) Experimental geometry and imaging scheme for FTH with the FZP first-order foci. The integrated mask contains both the object (1) to be imaged as well as a FZP (2). Positive and negative FZP diffraction orders are focused in a real and a virtual focal plane, respectively. The reference beams corresponding to these focal planes encode the phase information of the object beam by interference. In each focal plane, the object exit wave appears to be defocused by the FZP focal length f . ( b ) The Fourier transform of the recorded hologram is depicted on the left side, containing a defocused holographic object reconstruction (black box). A focused reconstruction can be obtained by numerically propagating the defocused reconstruction by ± f , yielding an in-focus image that is superimposed by the reconstruction of the opposite focal plane (middle). After defocusing the undesired opposite focal-plane contributions for both FZP diffraction orders, virtual and real-image reconstructions can be added to further improve the signal (right). Full size image Image reconstruction In the following, we describe our method on the basis of a first-order reconstruction as illustrated in Fig. 2 . The numerical propagation of the initial reconstruction ( R ) from the real focal plane ( n =1) back to the mask plane ( p = −f ) yields the desired focused object reconstruction, which is superimposed by the cross-correlations of the remaining defocused FZP orders with the object. The intense zero-order offset can be eliminated by a central beam block, effectively acting as a high-pass filter, which is widely used in diffractive imaging experiments to protect the charge-coupled device (CCD) or to sense small signals at high diffraction angles without saturating the detector in the centre. Attention should be drawn to the contribution of the reconstructions related to the remaining unfocused FZP diffraction orders n ≠0, in particular the contribution from the virtual FZP focus ( n = − 1). A similar problem is well known from in-line holography as the twin-image problem and several solutions have been proposed [29] , [30] , [31] , [32] . Methods requiring further measurements from reference beams or additional holograms recorded at different energy or distance are unsuitable for destructive single-shot imaging. Other methods are based on segmenting and erasing undesired on-axis reconstructions in their particular focal plane and imply some prior knowledge about the sample being investigated. Since the desired object reconstruction arises as a defocused superposition in the opposite focal plane, the erasure of the unwanted reconstruction in the respective focal plane causes a loss of desired object information and therefore results in artefacts. Here we introduce a new, few-cycle iterative method that does not require additional information about the sample or the reference beam from a priori knowledge or reference measurements, illustrated in Fig. 2 . Considering the reconstruction ( R −f ) propagated to p =− f , the most perturbing overlay ( R v −2f ) on the focused reconstruction ( R r 0 ) from the n= 1 focus is generated in the opposite (virtual) focal plane ( n =−1). This overlay image is defocused corresponding to a propagation distance of −2 f. A similar −2 f defocused image ( R r −2 f ) is part of the R − 3 f reconstruction obtained by propagating the specimen wave to the threefold focal distance p =−3 f , that is, R −3 f = R v −4 f +R r −2 f . Therefore, the −2 f defocused image is removed from the R −f reconstruction via calculation of the difference R −f − R − 3 f . This procedure gives a substantial improvement over the simple R −f reconstruction, since the perturbing virtual image is now defocused by −4 f instead of −2 f (and has negative sign). Similarly, by adding R − 5 f , the virtual image is further defocused to −6 f . 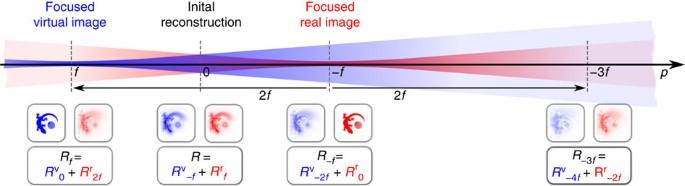Figure 2: Separating the first-order real image. The superposed virtual image contribution (Rv−2f) in the first-order reconstruction (R−f) can be gradually defocused by subtracting equivalently defocused real-image reconstructions at different propagation distancesp. Note that the propagated (cumulative) reconstructions (Rp) are indexed by the applied propagation distancep, while the individual contributions from the real image (RrΔp) and virtual image (RvΔp) have an index according to the displacement Δpfrom the respective focal plane. Consequently, an enhanced reconstruction ( R ′ − f ) can be obtained by gradually defocusing the undesired virtual image contribution: Figure 2: Separating the first-order real image. The superposed virtual image contribution ( R v −2 f ) in the first-order reconstruction ( R − f ) can be gradually defocused by subtracting equivalently defocused real-image reconstructions at different propagation distances p . Note that the propagated (cumulative) reconstructions ( R p ) are indexed by the applied propagation distance p , while the individual contributions from the real image ( R r Δ p ) and virtual image ( R v Δ p ) have an index according to the displacement Δ p from the respective focal plane. Full size image After a few iterations up to a certain maximum depth M , the disturbing background is sufficiently defocused and approaches a homogenous offset, that is, structure from the unwanted image is effectively removed. For contributions of higher FZP orders, this method can be repeated in a similar fashion. However, the impact of defocused higher-order superpositions in the reconstruction is much weaker since the diffraction efficiency of an ideal binary FZP drops with n −2 (ref. 19 ). In addition, the FZP focal length shortens for increasing diffraction orders, and contributions of higher orders are strongly defocused in a particular lower-order plane. We therefore restrict our attention exclusively to the first orders. Experimental demonstration To demonstrate our method, we have fabricated a sample ( Fig. 3a ) consisting of a 40-zone FZP with an outermost zone width of 50 nm, a conventional pinhole reference aperture and a test object. The test object comprises a gecko-shaped aperture surrounding a quadrant of a Siemens sector star, which allows evaluating the resolution achieved in the reconstruction. The conventional pinhole reference has a diameter of 60 nm, rendering the pinhole reconstruction directly comparable to the FZP-based FTH image. All objects are produced on a 100-nm-thick silicon nitride (Si 3 N 4 ) support membrane, which is coated by a 1-μm-thick gold film. In Fig. 3a , selected object features are presented as magnifications, including the geckos right feet (cyan, blue), an alignment hole closed by a deposited platinum dot (red) and some dirt grains (green, yellow) within the gecko object. The Pt deposit and the dirt grains are depicted from the Si 3 N 4 side where they are located. The gecko feet including the toes are shown from both sides. These features are not patterned completely through the entire gold mask thickness owing to the limited aspect ratio and the finite resolution achieved in fabrication via focused ion beam (FIB). The mask is illuminated with coherent synchrotron radiation of 400 eV photon energy and the recorded hologram is presented in Fig. 3b . The maximum momentum transfer recorded on the detector is 86 μm −1 and corresponds to a diffraction-limited resolution of 36 nm (half-period) in the reconstruction. The resolution of both pinhole and FZP reconstructions is therefore limited by the spatial extent of the reference structures. In Fig. 3c and d , we show the second quadrant of the Fourier-transformed hologram before and after numerical propagation of p =−1 f , respectively. To provide a uniform contrast of the different features in the overview figure, the reconstruction is high-pass filtered and depicted in logarithmic scale (amplitude). Apart from the central autocorrelation, the Fourier transform of the hologram consists of three contributions: ( R ) the cross-correlation of the FZP exit wave with the exit wave from the object, emerging as a superposition of defocused images related to all FZP foci, ( P o ) the cross-correlation of the exit waves of the pinhole and the object, and ( P FZP ) the pinhole reconstruction of the FZP. After numerically propagating the wave field by the FZP first-order focal length ( Fig. 3d ), P o appears defocused while P FZP shows a bright first-order focus. The desired reconstruction R is now focused but superposed by defocused reconstructions from all other FZP foci. The propagated FZP reconstruction without high-pass filtering is enlarged in Fig. 3e . The zeroth order is removed by suppressing low-frequency signals in the hologram with a Gauss function filter, and the sum of both filtered first-order reconstructions is shown in Fig. 3f . The final image is retrieved after applying M =5 iterations of our method to remove the associated image contribution in the opposite focal plane individually on both first-order reconstructions before summation ( Fig. 3g ). To demonstrate the efficiency of our method, holograms with different exposure times have been recorded, and the fully filtered FZP reconstructions are compared with the pinhole reconstructions in Fig. 4a . 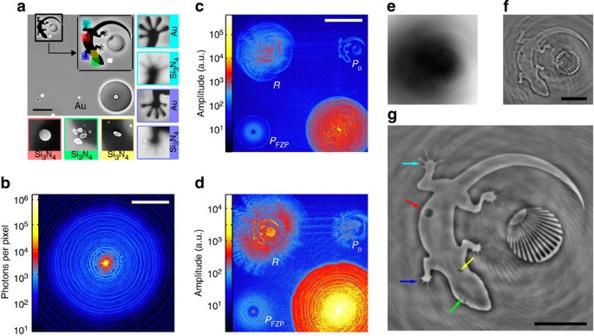Figure 3: High-resolution holography using an integrated zone plate reference. (a) Integrated mask with test object, conventional reference pinhole and FZP reference imaged by scanning electron microscopy (SEM) from the Au side of the sample (high dynamic range image to visualize features at front and back of the membrane). The bright squares and disks correspond to Pt deposits used to close alignment holes. These structures are opaque to soft X-rays. In the magnified inset (dimensions: 7 × 7 μm2), selected features of the object have been marked. SEM-imaged sections of these features with a size of 1 × 1 μm2were taken from the Si3N4or Au side as indicated. Scale bar, 5 μm distance. (b) Far-field X-ray diffraction pattern depicted in logarithmic intensity scale. Scale bar, 50 μm−1momentum transfer. (c) High-pass filtered holographic reconstruction (logarithmic amplitude) containing the cross-correlation of FZP and test object (R), the cross-correlation of test object and reference pinhole (PO), and the cross-correlation of reference pinhole and FZP (PFZP). Scale bar, 10 μm distance. (d) Holographic reconstruction after numerical propagation by the FZP focal length. (e) Cropped reconstruction of the desired image (real part) after numerical propagation by the FZP focal length. (f) The same image after removal of the zeroth order offset by high-pass filtering. Scale bar, 2 μm distance. (g) Image reconstruction after gradual defocusing the unwanted contribution from the opposite focal plane reconstruction. The arrows point to the features that were selected from SEM images in panela. Scale bar, 2 μm distance. Figure 3: High-resolution holography using an integrated zone plate reference. ( a ) Integrated mask with test object, conventional reference pinhole and FZP reference imaged by scanning electron microscopy (SEM) from the Au side of the sample (high dynamic range image to visualize features at front and back of the membrane). The bright squares and disks correspond to Pt deposits used to close alignment holes. These structures are opaque to soft X-rays. In the magnified inset (dimensions: 7 × 7 μm 2 ), selected features of the object have been marked. SEM-imaged sections of these features with a size of 1 × 1 μm 2 were taken from the Si 3 N 4 or Au side as indicated. Scale bar, 5 μm distance. ( b ) Far-field X-ray diffraction pattern depicted in logarithmic intensity scale. Scale bar, 50 μm −1 momentum transfer. ( c ) High-pass filtered holographic reconstruction (logarithmic amplitude) containing the cross-correlation of FZP and test object ( R ), the cross-correlation of test object and reference pinhole ( P O ), and the cross-correlation of reference pinhole and FZP (P FZP ). Scale bar, 10 μm distance. ( d ) Holographic reconstruction after numerical propagation by the FZP focal length. ( e ) Cropped reconstruction of the desired image (real part) after numerical propagation by the FZP focal length. ( f ) The same image after removal of the zeroth order offset by high-pass filtering. Scale bar, 2 μm distance. ( g ) Image reconstruction after gradual defocusing the unwanted contribution from the opposite focal plane reconstruction. The arrows point to the features that were selected from SEM images in panel a . Scale bar, 2 μm distance. 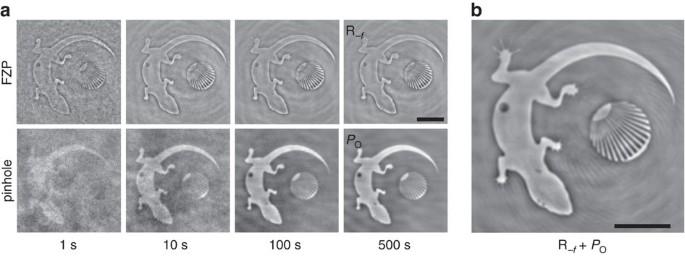Figure 4: Efficiency of the zone plate reference versus the pinhole reference. (a) The images show the reconstructions of our test object (real part) via the pinhole reference and the Fresnel zone plate (FZP) reference, obtained from the same holograms of the integrated mask (Fig. 2a) for different exposure times. Focused reference beam holographic images are reconstructed with our algorithm to remove contributions from the associated reconstruction in the opposite focal plane. The FZP reference reconstructions feature an improved signal-to-noise ratio and a higher spatial resolution. (b) Combined object reconstruction. In contrast toFigs 3dand5, low-frequency components of the object are now included via summation of pinhole and FZP reconstructions. Scale bars, 2 μm distance. Full size image Figure 4: Efficiency of the zone plate reference versus the pinhole reference. ( a ) The images show the reconstructions of our test object (real part) via the pinhole reference and the Fresnel zone plate (FZP) reference, obtained from the same holograms of the integrated mask ( Fig. 2a ) for different exposure times. Focused reference beam holographic images are reconstructed with our algorithm to remove contributions from the associated reconstruction in the opposite focal plane. The FZP reference reconstructions feature an improved signal-to-noise ratio and a higher spatial resolution. ( b ) Combined object reconstruction. In contrast to Figs 3d and 5 , low-frequency components of the object are now included via summation of pinhole and FZP reconstructions. Scale bars, 2 μm distance. Full size image Evidently, reconstructions of the FZP feature a significantly improved signal-to-noise ratio for short exposures and a superior spatial resolution due to the small FZP focal spot. The superior resolution in FZP reconstruction is also evident at the gecko’s right hind foot, which shows clearly resolved toes. Most of the other toes transmit the X-rays too faintly to be resolved. As an option, one can to some extent recover low-frequency components of the test object not present in the FZP reconstruction via a pixel-wise summation of the pinhole reconstruction containing low-frequency data and the FZP, as illustrated in Fig. 4b . The resolution limit for the pinhole and the FZP reconstruction is determined by evaluating the contrast of the sector star in the centre of the test object for different radii ( Fig. 5 ). The Rayleigh resolution limit [19] is found at 124 nm full period for the pinhole (62 nm feature size) and 92 nm (46 nm feature size) for the FZP reconstruction. By using state-of-the-art FZPs with outermost zone widths approaching 10 nm [16] and the possibility to utilize higher diffraction orders [33] , [34] , sub-10 nm spatial resolution will become accessible on this basis in FTH. In conclusion, monolithic focused reference beam X-ray holography enhances signal strength and resolution of FTH images even when employing rather primitive FZPs. In particular, the approach decouples the formation of image contrast from the spatial resolution. Focused reference beam X-ray holography is straightforward to implement and permits the application of easy-to-fabricate FZPs, that is, by FIB milling [35] . We provide a robust algorithm to remove image artefacts arising from the diffractive nature of the FZP lens, yielding high-quality images. We note that the energy dispersion of a FZP and the resulting spatial separation of foci from distinct photon energies opens the possibility to encode the spectral response of an object in a multi-colour experiment into a single hologram, even in a single-shot exposure. In conjunction with the possibility to holographically encode images of multiple samples [36] and dynamic processes [2] , [5] , [14] , we envision the approach to enable dynamic studies on the few-nanometre level in particular at coherent X-ray sources. 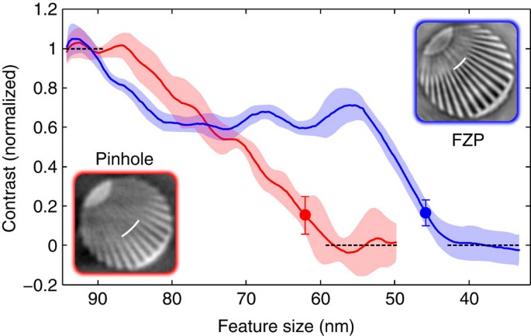Figure 5: Determination of image resolution. The plot shows the normalized image contrast in the sector star depending on the sector star’s line width for pinhole (red) and zone plate reconstruction (blue). Since the image background is not perfectly homogenous, the contrast is determined for the four central sectors (covered by the white arc) individually. The lines show the mean image contrast, whereas minima and maxima for normalization are obtained by averaging the contrast along the dashed lines. The confidence intervals according to the onefold s.d. of the contrast in the four different sectors are indicated by error bars and by the pale-coloured areas. The smallest resolvable feature sizes according to the Rayleigh resolution limit is determined with 62 nm (124 nm period) for the pinhole and 46 nm (92 nm period) for the FZP reconstruction (indicated by the points in the plot and by white arcs in the images). Figure 5: Determination of image resolution. The plot shows the normalized image contrast in the sector star depending on the sector star’s line width for pinhole (red) and zone plate reconstruction (blue). Since the image background is not perfectly homogenous, the contrast is determined for the four central sectors (covered by the white arc) individually. The lines show the mean image contrast, whereas minima and maxima for normalization are obtained by averaging the contrast along the dashed lines. The confidence intervals according to the onefold s.d. of the contrast in the four different sectors are indicated by error bars and by the pale-coloured areas. The smallest resolvable feature sizes according to the Rayleigh resolution limit is determined with 62 nm (124 nm period) for the pinhole and 46 nm (92 nm period) for the FZP reconstruction (indicated by the points in the plot and by white arcs in the images). Full size image Fabrication of the integrated mask The sample shown in Fig. 2a was fabricated on a Si 3 N 4 membrane coated on one side with a gold mask of 1 μm thickness. The FZP as well as the sector star pattern were generated by electron-beam lithography and subsequent electroplating of 30 nm Au on the opposite membrane side. The FZP has a diameter of 7.5 μm, 40 zones, and an outermost zone width of 50 nm. The sector star is 4 μm in diameter, comprises 64 periods and facilitates an evaluation of smallest resolvable feature sizes from 98 nm down to 23 nm (196–46 nm period). A FIB was used to mill a reference pinhole of 60 nm diameter and the gecko-shaped aperture as well as to unmask the FZP and the sector star. The apertures were positioned with the help of small alignment holes. After alignment, all alignment markers were closed by FIB-assisted deposition of 1 μm thick Pt dots on both membrane sides. The alignment hole located within the gecko aperture was closed from the Si 3 N 4 side only. In the scanning electron microscopic images in Fig. 3a , the deposited dots are visible as bright squares and disks. Experimental realization The experiment was performed at the UE52-SGM beamline of BESSY II in Berlin, Germany. The integrated mask was placed 170 mm downstream of the beamline focus and 325 mm in front of a back-illuminated, in-vacuum CCD camera (2,048 × 2,048 pixels) with pixels of 13.5 μm edge lengths. To increase the dynamic range of the holograms beyond the CCD limitations, a diffraction pattern recorded with a central beam stop was numerically combined with a diffraction pattern of the centre region, which was recorded by attenuating the incident X-ray beam with a gold filter of 150 nm thickness. How to cite this article: Geilhufe, J. et al . Monolithic focused reference beam X-ray holography. Nat. Commun. 5:3008 doi: 10.1038/ncomms4008 (2014).